Bacterial colonization dampens influenza-mediated acute lung injury via induction of M2 alveolar macrophages While the presence of airway bacteria is known to be associated with improved immunity against influenza virus, the mechanism by which endogenous microbiota influence antiviral immunity remains unclear. Here we show that specific pathogen-free mice are more sensitive to influenza-mediated death than mice living in a natural environment. Priming with Toll-like receptor 2-ligand + Staphylococcus aureus , which commonly colonizes the upper respiratory mucosa, significantly attenuates influenza-mediated lung immune injury. Toll-like receptor 2 deficiency or alveolar macrophage depletion abolishes this protection. S. aureus priming recruits peripheral CCR2 + CD11b + monocytes into the alveoli that polarize to M2 alveolar macrophages in an environment created by Toll-like receptor 2 signalling. M2 alveolar macrophages inhibit influenza-mediated lethal inflammation via anti-inflammatory cytokines and inhibitory ligands. Our results suggest a previously undescribed mechanism by which the airway microbiota may protect against influenza-mediated lethal inflammation. Under natural conditions, multiple bacterial species colonize the human upper respiratory mucosa and continually enter into the alveoli upon breathing. When this occurs, the pulmonary immune response to airway microbiota may influence the immune response to other ‘invader’ pathogens [1] , [2] , similar to the mechanism extensively described for gut microbiota [3] . Though commensal bacteria are crucial for maintaining intestinal immune homeostasis, as well as critical for protection against gut injury and associated mortality [3] , the role of airway microbiota in lung immune homeostasis is less well known. Previous studies have observed that secondary bacterial infections commonly cause additional mortality during influenza pandemics, suggesting that influenza-mediated immune suppression promotes pulmonary infection by bacteria [4] , [5] , [6] . On the other hand, some investigators demonstrated that commensal bacteria in the upper respiratory mucosa promote adaptive immunity against influenza virus by using antibiotics-treated mice [7] , [8] . This may partly explain why patients in developed countries, where the environment is relatively clean, have higher mortality and more severe disease than those in developing countries who may mount a stronger immune response to viral infection during influenza pandemics [9] . However, an alternative possibility is that the lung maintains a high threshold of immune ‘tolerance’ to avoid excessive inflammation by regulatory mechanisms, similar to the hygiene hypothesis in allergy [10] , [11] . Indeed, supporting this possibility, some pulmonary bacterial infections have been shown to attenuate anti-influenza virus inflammation [12] , [13] . Even though the evidence demonstrating a role for airway microbiota in inhibiting acute infectious inflammation has previously been reported, the immunological mechanisms underlying the interactions among the ‘invader’ influenza virus, ‘resident’ bacteria and host homeostasis have not been described. It has been noted that the predominant interactions between host and commensal bacteria are usually benign, and are often beneficial [14] . In our study, we observed that mice housed in a specific pathogen-free (SPF) environment are more sensitive to influenza-mediated death than mice living in a natural (non-SPF) environment when colonized in the upper respiratory tract by Toll-like receptor 2 (TLR2)-ligand + bacteria, including S. aureus . S. aureus is one of the most common commensal bacteria residing in the human upper respiratory tract; although ~25–50% of the human population are S. aureus carriers, the probability of S. aureus -induced pneumonia is relatively rare [15] . We therefore wanted to explore the physiological function of S. aureus in the upper respiratory tract by asking whether airway-colonized S. aureus , in a similar manner to intestinal commensal bacteria, have any role in lung immune homeostasis. In order to address this question, we generated a mouse model where the upper respiratory tract was commensally colonized with S. aureus , and observed that S. aureus priming protects mice against subsequent lethal influenza infection. We also show that CD11b + M2 alveolar macrophages (AMs), induced by continual TLR2 stimulation, are the major factors preventing influenza-mediated lethal inflammation. Thus, our data suggest that commensal bacteria in the airways may provide protection against lethal inflammation in the lung caused by influenza infection. S. aureus priming prevents influenza-mediated lung injury To examine how a changing environment influenced influenza-mediated pathology in the lung, we infected SPF mice and non-SPF mice intranasally (i.n.) with a lethal dose of the A/PR/8/34 (hereafter called PR8) influenza virus strain. Compared with SPF mice, non-SPF mice exhibited reduced body weight loss ( Fig. 1a ) and a higher survival rate ( Fig. 1b ). Furthermore, more bacteria were observed in the upper respiratory tract of non-SPF mice ( Fig. 1c ), suggesting that this protective effect may relate to increased commensal bacterial load. Surprisingly, we also found that non-SPF mice, but not SPF mice, were colonized by S. aureus among many other bacterial strains in the upper respiratory tract ( Fig. 1d , Supplementary Fig. S1 ). Using an established method reported in a previous study [16] , [17] , we used S. aureus as a tractable model for other unknown commensal bacteria, many of which are not tractable for these types of experiments, to construct a mouse model in which S. aureus commensally colonized the upper respiratory tract. We observed that S. aureus were detected in the upper respiratory tract but not in the lung 3 days after S. aureus priming ( Supplementary Fig. S2a,b ). At day 3 after S. aureus priming, there was no significant change between control mice and S. aureus -primed mice in body weight, physiological status of the lungs or total protein and inflammatory cytokine levels in bronchoalveolar lavage fluid (BALF) ( Supplementary Fig. S2c–f ), suggesting that the constructed mouse model could at least partly mimic the physiological status observed in S. aureus colonization of the upper respiratory tract. 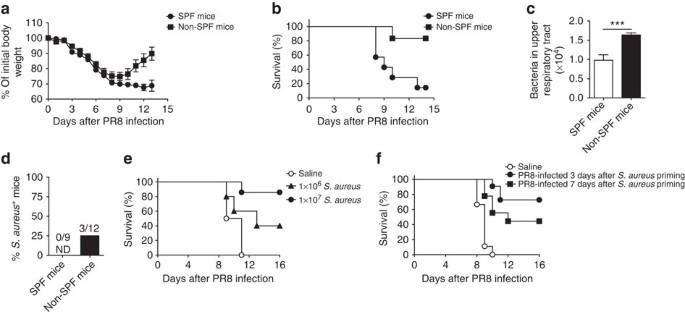Figure 1: Commensal bacteria protect mice against death mediated by influenza infection. (a) Change in body weight of mice housed in a SPF or non-SPF environment at the indicated times after infecting with a lethal dose (0.5 HA) of PR8. (b) Survival of SPF and non-SPF mice after infecting with 0.5 HA of PR8. (c) The number of bacteria in the upper respiratory tract of SPF and non-SPF mice. (d) The percentage of SPF and non-SPF mice colonized byS. aureusin the upper respiratory tract. (e) Three days after priming with control saline or with different doses ofS. aureus, WT mice were infected with 0.5 HA of PR8 and analysed for survival. (f) At the indicated time points after priming with 1 × 107CFU ofS. aureus, WT mice were infected with 0.5 HA of PR8 and analysed for survival. ND, not detected. Two-tailed Student’st-tests, ***P<0.001. Data are expressed as mean±s.e.m. Data represent three independent experiments with at least five mice per group in (a,e,f), or represent two independent experiments with at least five mice per group in (b–d). Figure 1: Commensal bacteria protect mice against death mediated by influenza infection. ( a ) Change in body weight of mice housed in a SPF or non-SPF environment at the indicated times after infecting with a lethal dose (0.5 HA) of PR8. ( b ) Survival of SPF and non-SPF mice after infecting with 0.5 HA of PR8. ( c ) The number of bacteria in the upper respiratory tract of SPF and non-SPF mice. ( d ) The percentage of SPF and non-SPF mice colonized by S. aureus in the upper respiratory tract. ( e ) Three days after priming with control saline or with different doses of S. aureus , WT mice were infected with 0.5 HA of PR8 and analysed for survival. ( f ) At the indicated time points after priming with 1 × 10 7 CFU of S. aureus , WT mice were infected with 0.5 HA of PR8 and analysed for survival. ND, not detected. Two-tailed Student’s t -tests, *** P <0.001. Data are expressed as mean±s.e.m. Data represent three independent experiments with at least five mice per group in ( a , e , f ), or represent two independent experiments with at least five mice per group in ( b – d ). Full size image Next, to examine the effects of ‘resident’ S. aureus on other ‘invader’ respiratory pathogens, S. aureus -primed mice were infected i.n. with a lethal dose of PR8. Compared with control mice, mice primed with either 1 × 10 6 or 1 × 10 7 colony forming unit (CFU) of S. aureus 3 days before a lethal PR8 dose exhibited a significantly increased protective effect against PR8-mediated death ( Fig. 1e ), and this S. aureus -mediated protection was effective even when given 7 days before PR8 infection ( Fig. 1f ). Immune-mediated pathology has been shown to be responsible for influenza-mediated death [18] , [19] . In order to observe the dynamic effect of S. aureus priming on subsequent influenza-mediated pathological injury over time, we infected S. aureus -primed mice with a sublethal dose of PR8. Compared with control mice, S. aureus -primed mice exhibited reduced body weight loss during PR8 infection ( Fig. 2a ). Control mice were characterized as exhibiting severe bronchopneumonia and interstitial pneumonitis after PR8 infection, but lungs from S. aureus -primed mice were only slightly inflamed ( Fig. 2b ). The levels of total protein, inflammatory cytokines (including interleukin (IL)-6, tumour-necrosis factor-α, IL-17, interferon-γ (IFN-γ) and granulocyte–macrophage colony-stimulating factor) and chemokines (including CCL2, CXCL1 and CCL5) in BALF were also lower in S. aureus -primed mice at day 7 after PR8 infection ( Fig. 2d ). Similarly, S. aureus -primed mice exhibited less lung immune injury compared with control mice during a lethal dose of PR8 infection ( Supplementary Fig. S3 ). Together, these data indicate that S. aureus priming attenuates lung immune injury that subsequently protects mice against death during influenza infection. 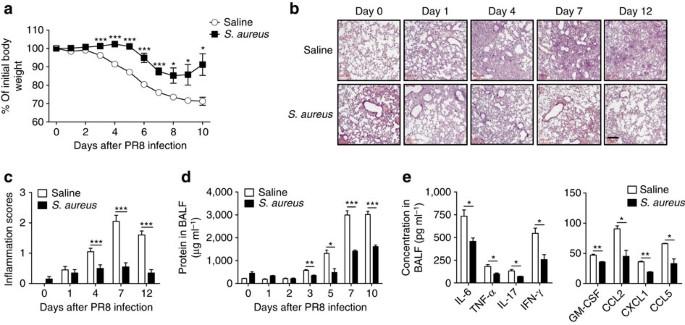Figure 2:S. aureuspriming attenuates lung injury mediated by influenza infection. (a) Change in body weight of control WT mice andS. aureus-primed WT mice at the indicated times after infecting with a sublethal dose (0.1 HA) of PR8. (b) Hematoxylin and eosin staining of lung, (c)inflammation scores and (d) BCA protein assay of total protein in BALF from control WT mice andS. aureus-primed WT mice at the indicated times after infecting with 0.1 HA of PR8. Scale bars represent 200 μm. (e) ELISA of cytokines and chemokines in BALF from control andS. aureus-primed WT mice at day 7 after infecting with 0.1 HA of PR8. Two-tailed Student’st-tests, *P<0.05, **P<0.01, ***P<0.001. Data are expressed as mean±s.e.m. Data represent three independent experiments with at least five mice per group in (a–e). Figure 2: S. aureus priming attenuates lung injury mediated by influenza infection. ( a ) Change in body weight of control WT mice and S. aureus- primed WT mice at the indicated times after infecting with a sublethal dose (0.1 HA) of PR8. ( b ) Hematoxylin and eosin staining of lung, ( c )inflammation scores and ( d ) BCA protein assay of total protein in BALF from control WT mice and S. aureus- primed WT mice at the indicated times after infecting with 0.1 HA of PR8. Scale bars represent 200 μm. ( e ) ELISA of cytokines and chemokines in BALF from control and S. aureus- primed WT mice at day 7 after infecting with 0.1 HA of PR8. Two-tailed Student’s t -tests, * P <0.05, ** P <0.01, *** P <0.001. Data are expressed as mean±s.e.m. Data represent three independent experiments with at least five mice per group in ( a – e ). Full size image Prevention of lung injury is TLR2-dependent TLR2 is important in activating the host immune response against S. aureus infection [20] . We therefore next tested whether TLR2 had a role in the S. aureus -induced prevention of influenza-mediated lung injury. Wild-type (WT) and Tlr2 −/− mice were primed with S. aureus 3 days before a lethal dose of PR8 influenza virus. Expectedly, S. aureus -primed Tlr2 −/− mice could not prevent PR8-mediated death, while S. aureus -primed Tlr4 −/− mice exhibited the same protective effect as S. aureus -primed WT mice ( Fig. 3a ). In addition, we compared the body weight changes and survival rates of non-SPF WT mice and non-SPF Tlr2 −/− mice after a lethal dose of PR8 infection and observed that although the non-SPF Tlr2 −/− mice had longer survival times than SPF WT mice after PR8 infection, it could not escape from influenza-mediated death as compared with non-SPF WT mice ( Supplementary Fig. S4 ). These data suggest that S. aureus -induced TLR2 activation is involved in this protective effect. Consistent with our finding, TLR2-ligand + Streptococcus pneumoniae priming has also been shown to protect mice against influenza-mediated death [21] , [22] . Moreover, WT, Tlr2 −/− and Tlr4 −/− mice infected with a lethal dose of PR8 alone exhibited no significant differences in mortality ( Supplementary Fig. S5a ), and Tlr2 −/− mice had the same ability to eliminate viruses or bacteria as WT mice ( Supplementary Fig. S5b,c ), suggesting that TLR2 deficiency did not directly influence mortality after lethal influenza infection. 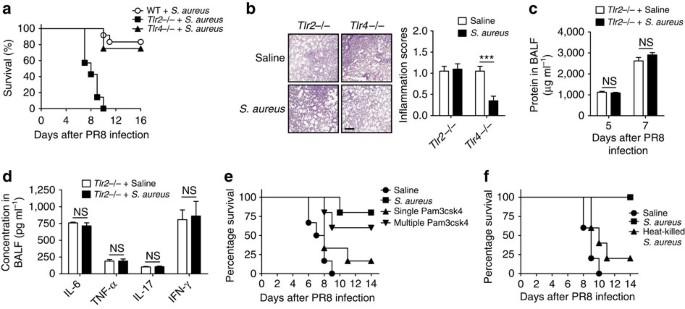Figure 3: TLR2 deficiency abolishesS. aureus-mediated prevention of influenza-mediated lung injury. (a) Three days afterS. aureuspriming, WT mice,Tlr2−/−mice andTlr4−/−mice were infected with 0.5 HA of PR8 and analysed for survival. (b) Hematoxylin and eosin staining and inflammation scores of the lungs from controlTlr2−/−andTlr4−/−mice andS. aureus-primedTlr2−/−andTlr4−/−mice at day 4 after infecting with 0.1 HA of PR8. Scale bars represent 200 μm. (c) BCA protein assay of total protein in BALF from controlTlr2−/−mice andS. aureus-primedTlr2−/−mice at days 5 and 7 after infecting with 0.1 HA of PR8. (d) ELISA of cytokines in BALF from controlTlr2−/−mice andS. aureus-primedTlr2−/−mice at day 7 after infecting with 0.1 HA of PR8. (e) Three days after priming WT mice with a single dose of Pam3csk4 (a TLR2 agonist), multiple Pam3csk4 doses (twice a day for 3 days), or 1 × 107CFU ofS. aureus,mice were then infected with 0.5 HA of PR8 and analysed for survival. (f) Three days after priming with 1 × 107CFU of either liveS. aureusor heat-killedS. aureus, WT mice were infected with 0.5 HA of PR8 and analysed for survival. Two-tailed Student’st-tests; NS, not significant; ***P<0.001. Data are expressed as mean±s.e.m. Data represent three independent experiments with at least five mice per group in (a–d), or represent two independent experiments with at least five mice per group in (e,f). Figure 3: TLR2 deficiency abolishes S. aureus -mediated prevention of influenza-mediated lung injury. ( a ) Three days after S. aureus priming, WT mice, Tlr2 −/− mice and Tlr4 −/− mice were infected with 0.5 HA of PR8 and analysed for survival. ( b ) Hematoxylin and eosin staining and inflammation scores of the lungs from control Tlr2 −/− and Tlr4 −/− mice and S. aureus- primed Tlr2 −/− and Tlr4 −/− mice at day 4 after infecting with 0.1 HA of PR8. Scale bars represent 200 μm. ( c ) BCA protein assay of total protein in BALF from control Tlr2 −/− mice and S. aureus- primed Tlr2 −/− mice at days 5 and 7 after infecting with 0.1 HA of PR8. ( d ) ELISA of cytokines in BALF from control Tlr2 −/− mice and S. aureus- primed Tlr2 −/− mice at day 7 after infecting with 0.1 HA of PR8. ( e ) Three days after priming WT mice with a single dose of Pam3csk4 (a TLR2 agonist), multiple Pam3csk4 doses (twice a day for 3 days), or 1 × 10 7 CFU of S. aureus, mice were then infected with 0.5 HA of PR8 and analysed for survival. ( f ) Three days after priming with 1 × 10 7 CFU of either live S. aureus or heat-killed S. aureus , WT mice were infected with 0.5 HA of PR8 and analysed for survival. Two-tailed Student’s t -tests; NS, not significant; *** P <0.001. Data are expressed as mean±s.e.m. Data represent three independent experiments with at least five mice per group in ( a – d ), or represent two independent experiments with at least five mice per group in ( e , f ). Full size image To explore how TLR2 promotes the protective effect of S. aureus priming on influenza-mediated lung injury, we infected S. aureus -primed Tlr2 −/− mice with a sublethal dose of PR8. Immunopathological analysis indicated that S. aureus priming did not attenuate PR8-mediated lung immune injury in Tlr2 −/− mice as compared with Tlr4 −/− mice ( Fig. 3b ). Furthermore, S. aureus priming did not decrease the levels of total protein ( Fig. 3c ) or inflammatory cytokines ( Fig. 3d ) in BALF from Tlr2 −/− mice after PR8 infection. To further demonstrate the role of TLR2 in the S. aureus -induced protective effect, we primed mice i.n. with TLR2 agonist, Pam3csk4, and then infected mice with PR8. While priming with a single treatment of Pam3csk4 or heat-killed S. aureus did not protect mice against PR8-mediated death, treating mice with multiple Pam3csk4 doses over several days was able to protect mice ( Fig. 3e ). Collectively, these data suggest that persistent TLR2 signalling is essential for S. aureus -induced protection against influenza-mediated death. Influenza-mediated death also correlates to high virus loads [23] . However, we found that S. aureus -primed WT and Tlr2 −/− mice harboured similar PR8 loads in the lungs during both sublethal and lethal dose of PR8 infection ( Supplementary Fig. S5d,e ), suggesting that S. aureus -mediated TLR2-dependent protection did not depend on inhibiting viral proliferation. Together, these data suggest that S. aureus -mediated TLR2-dependent protective effect depends on downregulating inflammation rather than inhibiting influenza virus replication. M2 AMs prevent influenza-mediated death As our data show that TLR2 is involved in preventing influenza-mediated death, we next explored which cells in the alveoli expressed TLR2 after S. aureus priming. TLR2 expression on AMs was upregulated after S. aureus priming ( Fig. 4a ). Given that AMs have been shown to be critical for maintaining immune homeostasis in the lungs [24] , we examined whether AMs were involved in the S. aureus -induced mechanism preventing influenza-mediated death. In our study, AMs could directly engulf green fluorescent protein-labelled S. aureus ( Supplementary Fig. S6 ), suggesting that S. aureus could interact with and activate the AMs. Consistent with these data, the number of AMs increased in the alveoli during the early stages of S. aureus priming ( Fig. 4b ). Next, to determine whether AMs were required, we treated mice i.n. with CL 2 MDP-lip to deplete AMs 2 days before S. aureus priming and observed that there were fewer AMs in BALF from CL 2 MDP-lip-treated mice at day 3 after S. aureus priming when compared with PBS-lip-treated mice ( Fig. 4c ). AM depletion did not directly affect elimination of either PR8 or S. aureus from the lung ( Supplementary Fig. S7a,b ). More importantly, in contrast to control PBS-lip-treated mice, S. aureus priming did not protect CL 2 MDP-lip-treated mice against PR8-mediated death ( Fig. 4d ). Further studies showed that adoptively transferring AMs from S. aureus -primed WT mice protected S. aureus -primed AM-depleted WT mice against PR8-mediated death and prolonged survival time of AM-depleted WT mice, AM-depleted Tlr2 −/− mice and S. aureus -primed AM-depleted Tlr2 −/− mice after PR8 infection. However, adoptively transferring AMs from control WT mice or S. aureus -primed Tlr2 −/− mice could not protect S. aureus -primed AM-depleted WT mice against PR8-mediated death ( Fig. 4e ). Taken together, these data suggested that only S. aureus priming in a TLR2-sufficient environment produce AMs that confer protection against influenza-mediated death. It further suggested that sustaining the AM-mediated protective effect also requires a lung environment created by TLR2 signalling. In addition, S. aureus -primed CL 2 MDP-lip-treated mice harboured similar PR8 loads in the lungs as PBS-lip-treated mice ( Supplementary Fig. S7c ). Therefore, these data indicate that AMs activated by S. aureus priming are involved in preventing influenza-mediated death without affecting viral load. 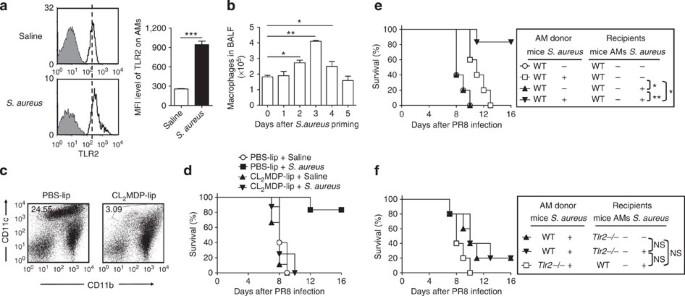Figure 4: Attenuation of influenza-mediated lung injury requires AMs duringS. aureuspriming. (a) Surface expression of TLR2 on AMs from WT mice at day 3 afterS. aureuspriming. (b) The number of AMs from WT mice at the indicated time points afterS. aureuspriming. (c) Two days after CL2MDP-lip treatment, mice were primed withS. aureusand then analysed for AMs in BALF 3 days later. (d) Three days after priming with control saline orS. aureus, control PBS-lip-treated and CL2MDP-lip-treated WT mice were infected with 0.5 HA of PR8 and analysed for survival. (e) Two days after CL2MDP-lip treatment, mice were primed with control saline orS. aureus, and then AMs from control orS. aureus-primed WT mice were adoptively transferred i.n. into these mice 3 days later. Survival of recipient mice was measured after infecting with 0.5 HA of PR8 immediately after adoptive transfer. (f) Two days after CL2MDP-lip treatment, mice were primed with control saline orS. aureus, and then AMs fromS. aureus-primed WT mice orS. aureus-primedTlr2−/−mice were adoptively transferred i.n. into these mice 3 days later. Survival of recipient mice was measured after infecting with 0.5 HA of PR8 immediately after adoptive transfer. Two-tailed Student’st-tests were used in (a,b), Gehan–Breslow–Wilcoxon tests were used in (e,f); NS, not significant; *P<0.05, **P<0.01, ***P<0.001. Data are expressed as mean±s.e.m. Data represent three independent experiments with at least five mice per group in (a–d), or represent two independent experiments with at least five mice per group in (e,f). Figure 4: Attenuation of influenza-mediated lung injury requires AMs during S. aureus priming. ( a ) Surface expression of TLR2 on AMs from WT mice at day 3 after S. aureus priming. ( b ) The number of AMs from WT mice at the indicated time points after S. aureus priming. ( c ) Two days after CL 2 MDP-lip treatment, mice were primed with S. aureus and then analysed for AMs in BALF 3 days later. ( d ) Three days after priming with control saline or S. aureus , control PBS-lip-treated and CL 2 MDP-lip-treated WT mice were infected with 0.5 HA of PR8 and analysed for survival. ( e ) Two days after CL 2 MDP-lip treatment, mice were primed with control saline or S. aureus , and then AMs from control or S. aureus -primed WT mice were adoptively transferred i.n. into these mice 3 days later. Survival of recipient mice was measured after infecting with 0.5 HA of PR8 immediately after adoptive transfer. ( f ) Two days after CL 2 MDP-lip treatment, mice were primed with control saline or S. aureus , and then AMs from S. aureus -primed WT mice or S. aureus -primed Tlr2 −/− mice were adoptively transferred i.n. into these mice 3 days later. Survival of recipient mice was measured after infecting with 0.5 HA of PR8 immediately after adoptive transfer. Two-tailed Student’s t -tests were used in ( a , b ), Gehan–Breslow–Wilcoxon tests were used in ( e , f ); NS, not significant; * P <0.05, ** P <0.01, *** P <0.001. Data are expressed as mean±s.e.m. Data represent three independent experiments with at least five mice per group in ( a – d ), or represent two independent experiments with at least five mice per group in ( e , f ). Full size image As S. aureus priming renders mice resistant to influenza-mediated death by attenuating lung immune injury, and AMs are involved in this process, we next examined whether AMs could inhibit influenza-mediated inflammation. The M2 macrophage has an immunosuppressive phenotype that can inhibit and resolve inflammation during infection [25] . In our study, S. aureus priming upregulated expression of the M2 macrophages surface markers, CD206 and Dectin-1 (ref. 26 ), on AMs ( Supplementary Fig. S8a ). In addition, expression of M2 macrophages-related genes [27] encoding Arg1, Ym1, Fizz1, IL-10 and TGF-β gradually increased in AMs from day 1 to day 3 after S. aureus priming ( Fig. 5a ). Meanwhile, iNOS gene expression, a marker of M1 macrophages, gradually decreased in AMs ( Fig. 5b ). Furthermore, AMs from S. aureus -primed WT mice exhibited the greatest inhibitory effect on Con A-stimulated T-cell proliferation in vitro ( Fig. 5c ). Therefore, these data suggest that S. aureus priming can induce AMs to polarize towards M2 phenotype cells, which are critical to attenuate lung immune injury mediated by influenza infection. 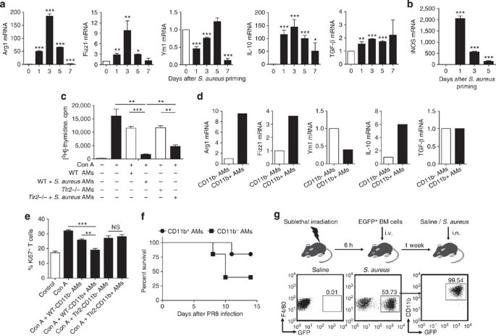Figure 5:S. aureussustains CD11b+M2 AM generation from non-resident monocyte. (a,b) Quantitative RT–PCR analysis of the expression of Arg1, Fizz1, Ym1, IL-10, TGF-β (a) and iNOS (b) mRNAs in AMs from WT mice at the indicated time points afterS. aureuspriming. (c) AMs from WT mice orTlr2−/−mice at day 3 afterS. aureuspriming were co-cultured with naïve splenocytes and stimulated by Con A; 3 days later, [3H]-thymidine incorporation in T cells was analysed. (d) Quantitative RT–PCR analysis of the expression of Arg1, Fizz1, Ym1, IL-10 and TGF-β mRNAs in CD11b−and CD11b+AMs from WT mice at day 3 afterS. aureuspriming. (e) CD11b−and CD11b+AMs from WT mice orTlr2−/−mice at day 3 afterS. aureuspriming were co-cultured with naïve splenocytes and stimulated by Con A; 3 days later, the expression of Ki67 in T cells was evaluated. (f) Two days after CL2MDP-lip treatment, WT mice were primed withS. aureus, and then CD11b−or CD11b+AMs fromS. aureus-primed WT mice were adoptively transferred i.n. into these mice 3 days later. Survival of recipient mice was measured after infecting with 0.5 HA of PR8 immediately after adoptive transfer. (g) Six hours after sublethal irradiation, 5 × 106EGFP+BM cells were adoptively transferred i.v. into WT mice and then primed withS. aureus7 days later. The percentage of EGFP+AMs in recipient mice at day 3 afterS. aureuspriming was evaluated by flow cytometry. Two-tailed Student’st-tests; NS, not significant; *P<0.05, **P<0.01, ***P<0.001. Data are expressed as mean±s.e.m. Data represent three independent experiments with at least five mice per group in (a,b), or represent two independent experiments with at least five mice per group in (f,g), or represent three independent experiments with three wells per treatment in (c,e). Figure 5: S. aureus sustains CD11b + M2 AM generation from non-resident monocyte. ( a , b ) Quantitative RT–PCR analysis of the expression of Arg1, Fizz1, Ym1, IL-10, TGF-β ( a ) and iNOS ( b ) mRNAs in AMs from WT mice at the indicated time points after S. aureus priming. ( c ) AMs from WT mice or Tlr2 −/− mice at day 3 after S. aureus priming were co-cultured with naïve splenocytes and stimulated by Con A; 3 days later, [ 3 H]-thymidine incorporation in T cells was analysed. ( d ) Quantitative RT–PCR analysis of the expression of Arg1, Fizz1, Ym1, IL-10 and TGF-β mRNAs in CD11b − and CD11b + AMs from WT mice at day 3 after S. aureus priming. ( e ) CD11b − and CD11b + AMs from WT mice or Tlr2 −/− mice at day 3 after S. aureus priming were co-cultured with naïve splenocytes and stimulated by Con A; 3 days later, the expression of Ki67 in T cells was evaluated. ( f ) Two days after CL 2 MDP-lip treatment, WT mice were primed with S. aureus , and then CD11b − or CD11b + AMs from S. aureus -primed WT mice were adoptively transferred i.n. into these mice 3 days later. Survival of recipient mice was measured after infecting with 0.5 HA of PR8 immediately after adoptive transfer. ( g ) Six hours after sublethal irradiation, 5 × 10 6 EGFP + BM cells were adoptively transferred i.v. into WT mice and then primed with S. aureus 7 days later. The percentage of EGFP + AMs in recipient mice at day 3 after S. aureus priming was evaluated by flow cytometry. Two-tailed Student’s t -tests; NS, not significant; * P <0.05, ** P <0.01, *** P <0.001. Data are expressed as mean±s.e.m. Data represent three independent experiments with at least five mice per group in ( a , b ), or represent two independent experiments with at least five mice per group in ( f , g ), or represent three independent experiments with three wells per treatment in ( c , e ). Full size image Normally, AMs exhibit a unique F4/80 hi CD11c hi CD11b − phenotype [28] . However, we found that a population of F4/80 hi CD11c hi CD11b + AMs appeared after S. aureus priming. To determine which AM population were M2 macrophages, we purified CD11b − and CD11b + AMs by cell sorting and found that CD206 and Dectin-1 expression ( Supplementary Fig. S8b ), as well as the expression of genes encoding Arg1, Fizz1 and IL-10 ( Fig. 5d ), were higher in CD11b + than in CD11b − AMs. Furthermore, CD11b + AMs from S. aureus -primed WT mice exhibited an enhanced inhibitory effect on Con A-stimulated T-cell proliferation in vitro compared with CD11b − AMs ( Fig. 5e ), and CD11b + AMs adoptively transferred into S. aureus -primed AM-depleted mice exhibited a better protective effect than CD11b − AMs in vivo ( Fig. 5f ). Therefore, these data suggest that M2 macrophages originate from F4/80 hi CD11c hi CD11b + AMs. During respiratory tract infections, peripheral blood monocytes are recruited into the alveoli to expand the AM population in the lung [29] . To determine whether the CD11b + AMs come from peripheral blood monocytes, we adoptively transferred EGFP + bone marrow cells intravenously (i.v.) into sublethally irradiated mice and then primed mice with S. aureus 7 days later. A large population of EGFP + macrophages in the AM population was detected 3 days after S. aureus priming, and almost all EGFP + macrophages were CD11b + . No EGFP + AMs were detected in control mice ( Fig. 5g ). Furthermore, high levels of the monocyte chemoattractant protein, CCL2, were detected in the lungs from WT mice, but not from Tlr2 −/− mice, after S. aureus priming ( Supplementary Fig. S9a ). Anti-CCL2 neutralizing antibody treatment significantly decreased the percentage and number of CD11b + AMs in the alveoli after S. aureus priming ( Supplementary Fig. S9b ), suggesting that circulating CCR2 + monocytes were recruited into the alveoli through CCL2-mediated chemotaxis during S. aureus priming. Taken together, these data suggest that CD11b + peripheral blood monocytes are recruited into the alveoli and then polarized to M2 AMs during S. aureus priming. Monocyte recruitment and polarization depend on TLR2 As TLR2 promoted the prevention of influenza-mediated death, we next examined whether TLR2 influenced the production or differentiation of M2 AMs. M2 polarization of macrophages depends on the presence of IL-4 or IL-13, and IFN-γ can inhibit this process [30] . We first tested WT mice and found that high IL-13 levels were detected in BALF at day 3 after S. aureus priming ( Fig. 6a ), but IL-4 and IFN-γ were not detected. Further studies indicated that NKT cells, but not CD4 + T, CD8 + T, NK or AM cells, may be the main source of IL-13 during S. aureus priming ( Supplementary Fig. S10 ). To confirm the effect of IL-13 on M2 AMs polarization in our model, we treated WT mice i.n. with a neutralizing anti-IL-13 antibody during S. aureus priming, and found that IL-13 neutralization inhibited M2 AMs polarization and abolished the protective effect against PR8-mediated lung injury and death ( Fig. 6b–d ). Therefore, S. aureus priming-induced IL-13 is critical for M2 AM polarization. When Tlr2 −/− mice were tested, we observed that IL-13 levels were reduced and fewer AMs in BALF were detected in Tlr2 −/− mice when compared with S. aureus -primed WT mice 3 day after S. aureus priming ( Fig. 6a ). Moreover, CD11b + AMs were also reduced in Tlr2 −/− mice after S. aureus priming ( Fig. 6f ). Furthermore, CD206 and Dectin-1 expression ( Supplementary Fig. S8c ), as well as expression of the genes encoding Arg1, Fizz1, IL-10 and TGF-β ( Fig. 6g ), were much lower in AMs from S. aureus -primed Tlr2 −/− mice than in S. aureus -primed WT mice. Together, these data suggest that an alveolar environment created by TLR2 signalling is essential for recruiting and polarizing peripheral blood monocytes to M2 AMs during S. aureus priming. 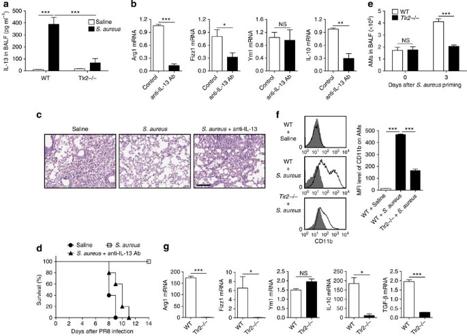Figure 6: The number of M2 AMs is decreased inTlr2−/−mice afterS. aureuspriming. (a) ELISA of IL-13 in BALF from WT mice andTlr2−/−mice at day 3 afterS. aureuspriming. (b) Quantitative RT–PCR analysis of the expression of Arg1, Fizz1, Ym1 and IL-10 mRNAs in AMs from control WT mice and anti-IL-13 neutralizing antibody-treated WT mice at day 3 afterS. aureuspriming. (c) Hematoxylin and eosin staining of the lungs from control mice,S. aureus-primed mice andS. aureus-primed anti-IL-13 neutralizing antibody-treated mice at day 5 after infecting with 0.5 HA of PR8. Scale bars represent 200 μm. (d) Survival of control mice,S. aureus-primed mice andS. aureus-primed anti-IL-13 neutralizing antibody-treated mice after infecting with 0.5 HA of PR8. (e) The number of AMs in BALF from WT mice andTlr2−/−mice at day 3 afterS. aureuspriming. (f) CD11b expression on AMs from WT mice andTlr2−/−mice at day 3 afterS. aureuspriming. (g) Quantitative RT–PCR analysis of the expression of Arg1, Fizz1, Ym1, IL-10 and TGF-β mRNA in AMs from WT mice andTlr2−/−mice at day 3 afterS. aureuspriming. Two-tailed Student’st-tests; NS, not significant; *P<0.05, **P<0.01, ***P<0.001. Data are expressed as mean±s.e.m. Data represent three independent experiments with at least five mice per group in (a,b,e–g), or represent two independent experiments with at least five mice per group in (c,d). Figure 6: The number of M2 AMs is decreased in Tlr2 −/− mice after S. aureus priming. ( a ) ELISA of IL-13 in BALF from WT mice and Tlr2 −/− mice at day 3 after S. aureus priming. ( b ) Quantitative RT–PCR analysis of the expression of Arg1, Fizz1, Ym1 and IL-10 mRNAs in AMs from control WT mice and anti-IL-13 neutralizing antibody-treated WT mice at day 3 after S. aureus priming. ( c ) Hematoxylin and eosin staining of the lungs from control mice, S. aureus -primed mice and S. aureus -primed anti-IL-13 neutralizing antibody-treated mice at day 5 after infecting with 0.5 HA of PR8. Scale bars represent 200 μm. ( d ) Survival of control mice, S. aureus -primed mice and S. aureus -primed anti-IL-13 neutralizing antibody-treated mice after infecting with 0.5 HA of PR8. ( e ) The number of AMs in BALF from WT mice and Tlr2 −/− mice at day 3 after S. aureus priming. ( f ) CD11b expression on AMs from WT mice and Tlr2 −/− mice at day 3 after S. aureus priming. ( g ) Quantitative RT–PCR analysis of the expression of Arg1, Fizz1, Ym1, IL-10 and TGF-β mRNA in AMs from WT mice and Tlr2 −/− mice at day 3 after S. aureus priming. Two-tailed Student’s t -tests; NS, not significant; * P <0.05, ** P <0.01, *** P <0.001. Data are expressed as mean±s.e.m. Data represent three independent experiments with at least five mice per group in ( a , b , e – g ), or represent two independent experiments with at least five mice per group in ( c , d ). Full size image M2 AMs inhibit inflammatory cells during influenza infection M2 macrophages can inhibit inflammation by secreting anti-inflammatory mediators and expressing inhibitory ligands [30] . Here, we observed that M2 AMs expressed high levels of the anti-inflammatory cytokines IL-10 and TGF-β after S. aureus priming in WT mice ( Fig. 5a ). To evaluate the effect of M2 AMs on influenza infection, we first confirmed that M2 AMs induced by S. aureus priming were also present during influenza infection, as the expression of genes encoding Arg1, Fizz1 and IL-10 in AMs from S. aureus- primed mice was higher than in AMs from control mice at day 3 after influenza infection. This significant difference disappeared by day 6 after PR8 infection ( Fig. 7a ), suggesting that M2 AMs might influence the early immune response against influenza infection. Indeed, further studies showed that while the number of macrophages was increased in S. aureus- primed mice during PR8 infection, the number of inflammatory cells, including NK cells and neutrophils, decreased ( Fig. 7b ). Moreover, S. aureus priming also decreased the number of CD8 + T cells in the alveoli in WT mice, but not in AM-depleted or Tlr2 −/− mice, during PR8 infection ( Fig. 7c ). To explore how AMs influence CD8 + T-cell proliferation, we evaluated T-cell subsets in the mediastinal lymph nodes (LNs) and found that the total cell number was decreased in mediastinal LNs from S. aureus- primed mice during PR8 infection ( Fig. 7d ), although CD4 + T and CD8 + T-cell proliferation capacity did not change ( Fig. 7e ). This result suggests that AMs might exert their primary function within the lung environment, and that AMs might influence T-cell proliferation in the mediastinal LNs in an indirect way. The inhibitory effect of M2 macrophages on T cells usually occurs through cell-to-cell contact in a PD-L1-dependent manner [31] . In our study, we found that S. aureus priming upregulates PD-L1 and PD-L2 expression on AMs ( Fig. 7f , Supplementary Fig. S11a ), and that both PD-L1 and PD-L2 expression are much higher on CD11b + M2 AMs than on CD11b − AMs ( Fig. 7g , Supplementary Fig. S11b ). Moreover, AMs from S. aureus- primed PR8-infected WT mice exhibit the greatest inhibitory effect on Con A-stimulated T-cell proliferation in vitro ( Fig. 7h ). Therefore, these data suggest that M2 AMs may function by inhibiting the recruitment and expansion of inflammatory cells to prevent mice from influenza-mediated death. 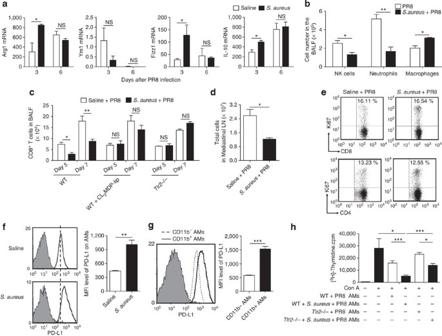Figure 7: M2 AMs decrease the number of inflammatory cells induced by influenza infection. (a) Quantitative RT–PCR analysis of the expression of Arg1, Fizz1, Ym1 and IL-10 mRNA in AMs from control andS. aureus-primed WT mice at days 3 and 6 after 0.1 HA of PR8 infection. (b) The number of NK cells, neutrophils and macrophages in BALF from control WT mice andS. aureus-primed WT mice at day 3 after infecting with 0.1 HA of PR8. (c) The number of CD8+T cells in BALF from control orS. aureus-primed WT, CL2MDP-lip-treated WT andTlr2−/−mice at days 5 and 7 after infecting with 0.1 HA of PR8. (d) The number of total cells in mediastinal LNs from control WT mice andS. aureus-primed WT mice at day 6 after infecting with 0.1 HA of PR8. (e) Ki67 expression in CD4+and CD8+T cells in mediastinal LNs from control WT mice andS. aureus-primed WT mice at day 6 after infecting with 0.1 HA of PR8. (f) PD-L1 expression on AMs from WT mice at day 3 afterS. aureuspriming. (g) PD-L1 expression on CD11b−and CD11b+AMs from WT mice at day 3 afterS. aureuspriming. (h) AMs fromS. aureus-primed WT orTlr2−/−mice at day 3 after influenza infection were co-cultured with naïve splenocytes and stimulated by Con A; 3 days later, [3H]-thymidine incorporation in T cells was analysed. Two-tailed Student’st-tests; NS, not significant; *P<0.05, **P<0.01, ***P<0.001. Data are expressed as mean±s.e.m. Data represent three independent experiments with at least five mice per group in (a–c,f,g), or represent two independent experiments with at least five mice per group in (d,e), or represent three independent experiments with three wells per treatment in (h). Figure 7: M2 AMs decrease the number of inflammatory cells induced by influenza infection. ( a ) Quantitative RT–PCR analysis of the expression of Arg1, Fizz1, Ym1 and IL-10 mRNA in AMs from control and S. aureus- primed WT mice at days 3 and 6 after 0.1 HA of PR8 infection. ( b ) The number of NK cells, neutrophils and macrophages in BALF from control WT mice and S. aureus- primed WT mice at day 3 after infecting with 0.1 HA of PR8. ( c ) The number of CD8 + T cells in BALF from control or S. aureus- primed WT, CL 2 MDP-lip-treated WT and Tlr2 −/− mice at days 5 and 7 after infecting with 0.1 HA of PR8. ( d ) The number of total cells in mediastinal LNs from control WT mice and S. aureus- primed WT mice at day 6 after infecting with 0.1 HA of PR8. ( e ) Ki67 expression in CD4 + and CD8 + T cells in mediastinal LNs from control WT mice and S. aureus- primed WT mice at day 6 after infecting with 0.1 HA of PR8. ( f ) PD-L1 expression on AMs from WT mice at day 3 after S. aureus priming. ( g ) PD-L1 expression on CD11b − and CD11b + AMs from WT mice at day 3 after S. aureus priming. ( h ) AMs from S. aureus -primed WT or Tlr2 −/− mice at day 3 after influenza infection were co-cultured with naïve splenocytes and stimulated by Con A; 3 days later, [ 3 H]-thymidine incorporation in T cells was analysed. Two-tailed Student’s t -tests; NS, not significant; * P <0.05, ** P <0.01, *** P <0.001. Data are expressed as mean±s.e.m. Data represent three independent experiments with at least five mice per group in ( a – c , f , g ), or represent two independent experiments with at least five mice per group in ( d , e ), or represent three independent experiments with three wells per treatment in ( h ). Full size image Commensal bacteria in the gut are important for maintaining intestinal immune homeostasis [32] . Various cellular components of these commensal bacteria in the gut can be recognized by TLRs to protect intestinal epithelium against gut injury and associated mortality. Under natural conditions, the human upper respiratory tract is also colonized by multiple commensal microbiota that may influence the respiratory immune system in a manner similar to the gut [3] . However, the role of airway microbiota in lung immune homeostasis is less well known, the key reason of which is lacking of the well-established animal model and enough experience. Accordingly, our study also faced this difficulty, but we improved the study system. In this report, we reveal that airway microbiota protects mice against influenza-mediated death, and this protective effect depends on attenuating immune injury rather than decreasing viral load ( Supplementary Fig. S12 ). So, our finding possibly provides a novel mechanism of how ‘resident’ airway bacteria maintain lung immune homeostasis to protect against ‘invader’ respiratory virus-mediated lethal inflammation. In contrast to our finding that airway bacteria negatively regulate the host immune response to viral infection, other studies found that airway microbiota promote and maintain host anti-virus immune response in respiratory mucosa. For example, antibiotic-treated mice display defective macrophage, CD4 + T-, CD8 + T- and B-cell immune responses when infected i.n. with the influenza virus [7] , [8] . However, we do not think that our results contradict these findings. As described for commensal gut bacteria, some bacteria are beneficial for maintaining intestinal homeostasis and health [33] , [34] , while others are likely to promote inflammation and disease [35] , [36] , [37] , [38] . Although the reason why commensal bacteria are associated with different immunological outcomes remains unclear, we speculate that the differing outcomes may be related to differences in the local pathophysiological condition in the lung, and more detailed studies are needed to address this idea. TLRs act as pattern recognition receptors (PRRs) that recognize pathogens and initiate innate immune responses. Among the TLRs, TLR2 is critical for sensing cellular components of S. aureus [20] . An interesting issue in our study is that TLR2 deficiency did not influence elimination of S. aureus , which was similar to the observation that MyD88 deficiency does not affect the elimination of S. aureus [39] ; this data imply that TLR2 is critical for lung homeostasis, but is not necessary for bacterial elimination. For the origin of AMs, previous studies have found that AMs can be derived primarily from peripheral blood monocytes, although a significant percentage of AMs are probably also originated from a self-renewing population of progenitor cells [40] , [41] , [42] . Interestingly, AMs have been noted previously as CD11b-negative, although CD11b expression is uniformly high on all other macrophage populations [43] . In our study, priming with commensal bacterium S. aureus recruited peripheral blood CD11b + monocytes into the alveoli, which are often considered as inflammatory monocytes during influenza infection [44] . The recruitment and function of inflammatory monocytes commonly happened in the early stage of influenza infection [44] , but CD11b + monocytes recruited by S. aureus priming in our study could maintain a long time to exert immune regulatory function and protect mice against subsequent influenza-mediated lung immune injury and death. Therefore, the CD11b + monocytes recruited by commensal bacterium S. aureus may be another macrophage population different from inflammatory monocytes reported previously in influenza infection. However, because the process how peripheral blood monocytes differentiate into AMs is still unclear until now [40] , [41] , [42] , the correlation between resident AMs and S. aureus priming-recruited CD11b + monocytes remains unclear. An analysis of the global 2009 H1N1 influenza epidemiology indicated that developed counties had higher morbidity and mortality rates as compared with developing countries [9] , [45] , which manifests similarly as what observed in allergy described by ‘hygiene hypothesis’. The observations in allergy and possibly in acute influenza infection supply a possibility that people living in developed countries (that is, in ‘clean’ environments) may be more sensitive, or may overreact, to influenza infection than people living in developing countries (that is, in ‘squalid’ environments). From our study, one possible explanation for this difference may be supplied that people in developing countries may harbour more commensal bacteria in their respiratory tracts, which can prime the local immune system and keep lung homeostasis when facing influenza attack. Mouse model of bacterial and viral infection The study involved animal experiments that were conducted ethically in accordance with the University of Science and Technology of China’s guidelines for the use and care of animals. Male C57BL/6 (B6) wild-type (WT) mice were purchased from the Shanghai Experimental Animal Center, Chinese Science Academy (Shanghai, China). Male Tlr2 −/− , Tlr4 −/− and EGFP-transgenic mice on the B6 background were bred in SPF conditions according to the experimental animal guidelines of the University of Science and Technology of China. For influenza infection studies, mice were anesthetized and infected i.n. with the A/PR/8/34 influenza virus strain (H1N1, PR8; lethal dose, 0.5 HA; sublethal dose, 0.1 HA) in 50 μl sterile saline. For S. aureu- priming studies, mice were anesthetized and primed i.n. with S. aureus (NCTC-8325 strain) in 50 μl sterile saline. For co-infection studies, mice were infected with PR8 at day 3 or day 7 after S. aureus priming. For Pam3csk4 (InvivoGen) treatment, mice in the single-treatment group received 15 μg Pam3csk4 i.n., and mice in the multiple-treatment group received 7.5 μg Pam3csk4 i.n. twice a day for 3 days. Twenty-four hours after the last Pam3csk4 treatment, mice were infected with PR8. For anti-IL-13 antibody (R&D) treatment, 60 μg was instilled i.n. into mice at days 0 and 2 during S. aureus priming. For anti-CCL2 antibody (Biolegend) treatment, 60 μg was injected i.v. into mice at day 0 during S. aureus priming. Determination of viral load Viral load in the lungs was determined by quantitative reverse transcriptase PCR (RT–PCR) analysis at the indicated time point after PR8 infection. Briefly, total RNA was extracted from whole lung tissue and then complementary DNA was synthesized. The viral load in each sample was calculated by relative quantification, and the ratio of viral RNA to β-actin messenger RNA at day 1 after PR8 infection in WT mice was used as a control. Primers ( Supplementary Table S1 ) were specific for the matrix protein of the influenza virus [46] . Quantification of bacterial burden To quantify the bacterial burden in the lungs at days 1, 2 and 3 after S. aureus priming, mice were killed and lung tissue was aseptically removed. Whole lung tissue was homogenized in 10 ml of sterile saline, and the tissue homogenate was serially diluted in sterile saline and then plated on blood agar. After 24-h incubation at 37 °C, colonies were counted, and CFUs per lung were determined. To quantify the commensal bacteria burden in the upper respiratory tract, nasal washes were collected by back-flushing 2 ml of sterile saline from the posterior nasopharyngeal opening, and plated with serial dilution as above [7] . Histopathology and inflammation scores Lung tissues were fixed in 10% neutral-buffered formalin for more than 24 h, embedded into paraffin and cut into 5-μm sections. Lung sections were stained with hematoxylin and eosin to determine histological changes. Twenty fields from right and left of the lung sections were randomly selected to determine inflammation scores according to a previously established scoring system [47] . Protein and cytokine measurement in BALF and lung homogenate BALF were collected by washing the lung once with 1 ml of sterile saline through an intratracheal cannula [12] , and whole lung tissue was homogenized in 10 ml sterile saline. The BCA protein assay Kit (Pierce, USA) was used for assaying the level of total protein in BALF. ELISA kits (Senxiong, China) were used to assay the levels of IL-4, IL-6, IL-13, IL-17, tumour-necrosis factor-α, IFN-γ, IL-1β, granulocyte–macrophage colony-stimulating factor, CCL2, CXCL1 and CCL5 in BALF. Cell recovery and AM isolation The lung was washed three times with 1 ml of 1 mM EDTA in DMEM through an intratracheal cannula. After centrifugation, the pellet was resuspended in DMEM (containing 10% FCS, penicillin (100 U ml −1 ), streptomycin (100 U ml −1 ) and 2 mM L -glutamine). For RNA extraction, AMs were isolated by adhering BAL cells to plastic for 1 h at 37 °C in 5% CO 2 (ref. 28 ). For adoptive transfer and in vitro culture experiments, AMs were sorted by flow cytometry (F4/80 hi CD11c hi ). The purity of AMs was over 95%. Quantitative RT–PCR analysis Quantitative RT–PCR analysis was performed according to the manufacturer’s instructions using a SYBR Premix Ex Taq (Takara). For analysis, the expression of target genes was normalized to the housekeeping gene β-actin. Gene expression values were calculated by using the mean of the samples from saline-treated mice as a calibrator. All primers ( Supplementary Table S1 ) were synthesized by Sangon Biotech (China). Flow cytometry assay After blocking the Fc receptor, single-cell suspensions were incubated with the indicated fluorescently labelled mAbs at 4 °C for 30 min in PBS (containing 0.1% sodium azide and 1% BSA), and then washed twice. For intracellular cytokine staining, cells were stimulated for 4 h at 37 °C with 50 ng ml −1 PMA, 1 μg ml −1 ionomycin and 10 μg ml −1 monensin (all from Sigma). After extracellular markers were stained, cells were fixed, permeabilized and stained with PE-anti-IL-13 or isotype control. Samples were analysed by BD LSR II and WINMDI2.9 software. All antibodies ( Supplementary Table S2 ) were from BD Biosciences, eBioscience, R&D or AbD Serotec. AM depletion and transfer AMs were depleted by treating i.n. with 100 μl Cl 2 MDP-Lip 48 h before priming (PBS-Lip was used as control) [4] , resulting in an ~90% decrease in AM number. For adoptive transfer studies, AM-depleted recipient mice were primed with S. aureus or saline. Three days later, 2 × 10 5 donor AMs from S. aureus -primed C57BL/6 or Tlr2 − / − mice were adoptively transferred i.n. into recipient mice, and the recipient mice were immediately infected with a lethal dose of PR8. EGFP + bone marrow (BM) cell transfer BM cells were isolated from EGFP-transgenic mice and resuspended in pyrogen-free PBS. C57BL/6 mice were irradiated with a sublethal doses (6 Gy for 3 min), and 5 × 10 6 EGFP + BM cells per mouse were adoptively transferred i.v. 6 h later. Seven days later, recipient mice were primed with S. aureus , and EGFP + AMs in BALF were detected by flow cytometry assay 3 days after S. aureus priming. Co-culture experiments and [ 3 H]-thymidine incorporation assay AMs were obtained by sorting cells from S. aureus- primed or S. aureus and PR8-coinfected C57BL/6 or Tlr2 −/− mice. For co-culture studies, AMs were seeded into 24-well cell culture plates at 2 × 10 5 cells per well along with 1.2 × 10 6 cells per well splenocytes from naïve C57BL/6 mice, and stimulated with 5 μg ml −1 Con A (Sigma-Aldrich) and 100 U ml −1 human recombinant IL-2 (Kingsley Pharmaceutical). After a 56-h incubation, 5 μCi ml −1 [Methyl- 3 H]-thymidine was added into the co-culture system, non-adherent cells were harvested 16 h later and the level of [Methyl- 3 H]-thymidine incorporation was determined. Statistical analysis Two-tailed Student’s t -tests were used for all other statistical analyses, except Gehan–Breslow–Wilcoxon tests were used for survival curve statistical analyses. The data were expressed as means±s.e.m. P <0.05 was considered statistically significant. How to cite this article: Wang, J. et al . Bacterial colonization dampens influenza-mediated acute lung injury via induction of M2 alveolar macrophages. Nat. Commun. 4:2106 doi: 10.1038/ncomms3106 (2013).